Activation of E-prostanoid 3 receptor in macrophages facilitates cardiac healing after myocardial infarction Two distinct monocyte (Mo)/macrophage (Mp) subsets (Ly6C low and Ly6C high ) orchestrate cardiac recovery process following myocardial infarction (MI). Prostaglandin (PG) E 2 is involved in the Mo/Mp-mediated inflammatory response, however, the role of its receptors in Mos/Mps in cardiac healing remains to be determined. Here we show that pharmacological inhibition or gene ablation of the Ep3 receptor in mice suppresses accumulation of Ly6C low Mos/Mps in infarcted hearts. Ep3 deletion in Mos/Mps markedly attenuates healing after MI by reducing neovascularization in peri-infarct zones. Ep3 deficiency diminishes CX3C chemokine receptor 1 (CX3CR1) expression and vascular endothelial growth factor (VEGF) secretion in Mos/Mps by suppressing TGFβ1 signalling and subsequently inhibits Ly6C low Mos/Mps migration and angiogenesis. Targeted overexpression of Ep3 receptors in Mos/Mps improves wound healing by enhancing angiogenesis. Thus, the PGE 2 /Ep3 axis promotes cardiac healing after MI by activating reparative Ly6C low Mos/Mps, indicating that Ep3 receptor activation may be a promising therapeutic target for acute MI. Healing of the infarcted myocardium involves a complex and coordinated process of inflammation, angiogenesis and tissue remodelling. Monocytes (Mos) and macrophages (Mps) in the infarcted myocardium are the essential immune cells for determining the progression and resolution of inflammation and repair following myocardial infarction (MI) [1] . Disruption of the Mo/Mp-mediated inflammatory response by Mo/Mp depletion or inhibition of Mo/Mp migration impairs wound healing and deteriorates left ventricular remodelling after MI [2] , [3] , [4] . In contrast, controlled activation of Mos/Mps ameliorates cardiac function and post MI remodelling by inducing Mo/Mp infiltration and neovascularization [5] . Two distinct subpopulations of Mos/Mps are involved in recovery after MI in a sequential pattern. Early responding Mos/Mps (Ly6C high ) are predominant 1–3 days after MI and display phagocytic and pro-inflammatory properties highly expressing tumour necrosis factor (TNF) α, interleukin (IL-6), myeloperoxidase, and cathepsins, whereas late-responding Mos/Mps (Ly6C low ) appear 4–7 days after MI and exhibit anti-inflammatory characteristics to support tissue regeneration by secreting reparative cytokines, such as IL-10, transforming growth factor (TGF) β1, and vascular endothelial growth factor (VEGF) [6] . Injured hearts express a unique chemokine profile over time to coordinate Mo recruitment, and the sequential recruitment of Ly6C high and Ly6C low Mos is dependent on C–C chemokine receptor type 2 (CCR2) and CX3C chemokine receptor 1 (CX3CR1), respectively [6] . Moreover, Ly6C high Mos can convert to Ly6C low Mos in circulation [7] , [8] and inflamed tissues including infarcted hearts [9] , [10] . Delayed transition of Ly6C high (M1-like) to Ly6C low Mos/Mps (M2-like), such as in atherosclerotic or diabetic animals [11] , [12] , attenuates wound repair post MI. Thus, targeting certain Mos/Mps as a therapeutic strategy for infarct healing and repair continues to receive intensive attention [13] . Prostaglandin (PG) E 2 is a key lipid mediator in many pathophysiological processes, including inflammation and immune responses, and it elicits diverse functions by acting on its four different E-prostanoid receptors (Ep1–Ep4) in a paracrine and autocrine manner [14] . Microsomal PGE 2 synthase-1 (mPGES-1), an inducible terminal isomerase for PGE 2 biosynthesis, is the major source of PGE 2 formed in vivo and during inflammatory responses [15] . Disabling PGE 2 generation by mPGHS-1 deletion leads to increased infarct sizes and adverse left ventricular remodelling after MI in mice [16] . Interestingly, mice with mPGES-1 deletion in bone marrow-derived myeloid cells alone displayssimilar cardiac phenotypes in global mPGES-1-deficient mice as subjected to coronary ligation [17] , strongly implicating Mos/Mps-derived PGE 2 in wound healing after MI. However, the underlying mechanisms are largely unknown. In this study, we investigated the role of PGE 2 receptors on recruitment of Mo/Mp subsets during inflammation and further explored effects of genetic deletion or overexpression of Ep3 receptor in Mos/Mps on cardiac healing in mice after acute MI. We found, disruption of Ep3 receptor in Mos/Mps resulted in augmented infarct size and reduced cardiac functions after MI through suppression of reparative Ly6C low infiltration and its mediated angiogenesis in peri-infarct zones in mice. Moreover, Ep3 deficiency in Mos/Mps inhibited TGFβ1 signalling to directly suppress transcription of Cx3cr1 and Vegf genes, therefore, retarding Ly6C low migration and neovascularization in the infarcted hearts. Controlled activation of Ep3 receptor in Mos/Mps facilitated Ly6C low infiltration and subsequent healing of MI by activation of TGFβ1 signalling. Thus, PGE 2 /Ep3 axis facilites cardiac healing after MI by activating reparative Ly6C low Mos/Mps. Ep3 mediates recruitment of Ly6C low Mos/Mps in peritonitis To explore which PGE 2 receptor subtype(s) mediate Mo/Mp recruitment in zymosan-induced peritonitis in mice, both Ly6C high and Ly6C low Mos/Mps were sorted by flow cytometry ( Fig. 1a ). Western blot analysis confirmed that the surface markers CCR2 and CX3CR1 were abundantly expressed in Ly6C high and Ly6C low cells, respectively ( Supplementary Fig. 1a ), and reverse transcriptase polymerase chain reaction (RT-PCR) showed that more pro-inflammatory genes were expressed in Ly6C high cells, while more reparative cytokines were expressed in Ly6C low cells ( Supplementary Fig. 1b,c ). All PGE 2 receptors ( Ep1–4 ) were differentially expressed in both Ly6C high and Ly6C low Mos/Mps, and Ly6C low Mos/Mps expressed more Ep1 and Ep3 receptors than Ly6C high Mos/Mps ( Fig. 1b ). Interestingly, the Ep3 receptor inhibitor L-798,106 reduced peritoneal infiltration of Ly6C low and total Mos/Mps without significantly influencing Ly6C high Mos/Mps, while the Ep1 receptor inhibitor SC-51322 retarded recruitment of Ly6C high Mos/Mps 48 h after the zymosan challenge ( Fig. 1c–e ). Consistently, L-798,106 significantly suppressed expression of reparative and pro-angiogenic cytokines ( IL-13, TGFβ1, VEGF and MMP9 ) and CX3CR1 in infiltrated Mos/Mps ( Fig. 1f ) without markedly altering expression of pro-inflammatory cytokines ( Fig. 1g ). In addition, by using myeloid cell-specific Ep3-deficient mice ( Ep3 F/F ;LysM Cre , Fig. 2a ), we also found Ep3 deficiency in Mos/Mps ( Fig. 2b ) markedly reduced total peritoneal Mos/Mps by restraining infiltration of Ly6C low Mos/Mps in response to a zymosan challenge in mice ( Fig. 2c–e ). Similarly, Ep3 deletion downregulated reparative cytokines and CX3CR1 gene expression in Mos/Mps without overt effects on the expression of the pro-inflammatory cytokines tested ( Fig. 2f,g ). 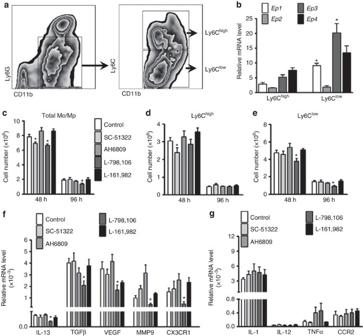Figure 1: Ep3 blockade represses recruitment of Ly6ClowMos/Mps in peritonitis in mice. (a) Gating strategy for peritoneal Ly6Chighand Ly6ClowMos/Mps in zymosan-induced peritonitis in mice. (b) Relative mRNA levels of the PG E2receptors (Ep1–4) in peritoneal Ly6Chighand Ly6ClowMos/Mps; data represent mean±s.e.m. *P<0.05 versus Ly6ChighMos/Mps (unpaired two-tailedt-test);n=5. (c–e) Effect of administration of different PGE2receptor blockers on recruitment of total Mos/Mps (c), Ly6Chigh(d), and Ly6Clow(e) Mos/Mps at 48 h and 96 h after a zymosan challenge in mice. Data represent mean±s.e.m. *P<0.05 versus control(unpaired two-tailedt-test);n=5–6. SC-51322,Ep1inhibitor; AH6809,Ep2inhibitor; L-798106,Ep3inhibitor; L-161982,Ep4inhibitor. (f,g) Effect of different PGE2receptor blockers on expression of anti-inflammatory (f) and pro-inflammatory (g) markers in peritoneal Mos/Mps collected 48 h after zymosan treatment. Data represent mean±s.e.m. *P<0.05 versus control (unpaired two-tailedt-test);n=4. Figure 1: Ep3 blockade represses recruitment of Ly6C low Mos/Mps in peritonitis in mice. ( a ) Gating strategy for peritoneal Ly6C high and Ly6C low Mos/Mps in zymosan-induced peritonitis in mice. ( b ) Relative mRNA levels of the PG E 2 receptors ( Ep1–4 ) in peritoneal Ly6C high and Ly6C low Mos/Mps; data represent mean±s.e.m. * P <0.05 versus Ly6C high Mos/Mps (unpaired two-tailed t- test); n =5. ( c – e ) Effect of administration of different PGE 2 receptor blockers on recruitment of total Mos/Mps ( c ), Ly6C high ( d ), and Ly6C low ( e ) Mos/Mps at 48 h and 96 h after a zymosan challenge in mice. Data represent mean±s.e.m. * P <0.05 versus control(unpaired two-tailed t -test); n =5–6. SC-51322, Ep1 inhibitor; AH6809, Ep2 inhibitor; L-798106, Ep3 inhibitor; L-161982, Ep4 inhibitor. ( f , g ) Effect of different PGE 2 receptor blockers on expression of anti-inflammatory ( f ) and pro-inflammatory ( g ) markers in peritoneal Mos/Mps collected 48 h after zymosan treatment. Data represent mean±s.e.m. * P <0.05 versus control (unpaired two-tailed t -test); n =4. 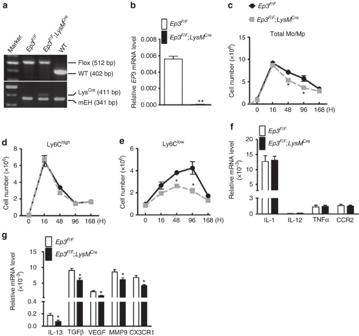Figure 2:Ep3deletion suppresses Ly6ClowMo/Mp infiltration in peritonitis in mice. (a) Genotyping ofEp3F/F;LysMCremice. Microsomal epoxide hydrolase (mEH) was used as quality control for extracted DNA from mouse tail biopsy. (b)Ep3receptor expression levels in peritoneal Mps fromEp3F/F;LysMCreandEp3F/Fmice. Data represent mean±s.e.m. **P<0.01 versusEp3F/F(unpaired two-tailedt-test);n=10. (c–e) Effect ofEp3deletion on recruitment of total Mos/Mps (c), Ly6Chigh(d), and Ly6Clowsubtype (e) Mos/Mps 48 and 96 h after a zymosan challenge in mice. Data represent mean±s.e.m. *P<0.05 versusEp3F/F(unpaired two-tailedt-test);n=5–7. (f,g) Effect ofEp3deficiency on expression of proinflammatory (f) and reparative angiogenic markers (g) in peritoneal Mos/Mps collected 48 h after zymosan treatment. Data represent mean±s.e.m. *P<0.05 versusEp3F/F(unpaired two-tailedt-test);n=10–11. Full size image Figure 2: Ep3 deletion suppresses Ly6C low Mo/Mp infiltration in peritonitis in mice. ( a ) Genotyping of Ep3 F/F ;LysM Cre mice. Microsomal epoxide hydrolase (mEH) was used as quality control for extracted DNA from mouse tail biopsy. ( b ) Ep3 receptor expression levels in peritoneal Mps from Ep3 F/F ;LysM Cre and Ep3 F/F mice. Data represent mean±s.e.m. ** P <0.01 versus Ep3 F/F (unpaired two-tailed t -test); n =10. ( c – e ) Effect of Ep3 deletion on recruitment of total Mos/Mps ( c ), Ly6C high ( d ), and Ly6C low subtype ( e ) Mos/Mps 48 and 96 h after a zymosan challenge in mice. Data represent mean±s.e.m. * P <0.05 versus Ep3 F/F (unpaired two-tailed t -test); n =5–7. ( f , g ) Effect of Ep3 deficiency on expression of proinflammatory ( f ) and reparative angiogenic markers ( g ) in peritoneal Mos/Mps collected 48 h after zymosan treatment. Data represent mean±s.e.m. * P <0.05 versus Ep3 F/F (unpaired two-tailed t -test); n =10–11. Full size image We then examined the effect of Ep3 deletion on the differentiation of recruited Mos in zymosan-induced peritonitis in mice. By day 1 after adoptive transfer ( Supplementary Fig. 2a ), ≈30% of the accumulated Ly6C high Mos had Ly6C low marker ( Supplementary Fig. 2b ), while Ep3 deficiency did not significantly influence Ly6C high Mo infiltration ( Supplementary Fig. 2c ) and its differentiation toward Ly6C low Mos/Mps ( Supplementary Fig. 2d ). In contrast, deletion of Ep3 receptor markedly reduced infiltration of Ly6C low Mos/Mps in zymosan-challenged peritoneal cavity ( Supplementary Fig. 2e,f ). Taken together, these results suggest that the Ep3 receptor is involved in mediating the recruitment of Ly6C low Mos/Mps in response to inflammatory insults. Ep3 promotes cardiac recovery by recruiting Ly6C low Mo/Mp Two Mo/Mp subsets (Ly6C low and Ly6C high ) are also implicated in recovery after MI—a sterile inflammatory reaction [6] . We then examined the role of Mo/Mp in cardiac repair after ischaemia in mice. As expected, all PG products, including PGE 2 , were elevated in infarcted hearts, although Ep3 deficiency in Mos/Mps had no significant influence on PG production ( Supplementary Fig. 3a–e ). CD11b + Ly6G − CD115 + Mos/Mps were sorted from infarcted hearts in mice ( Fig. 3a ). Notably, total infiltrated Mos/Mps in hearts were significantly reduced in Ep3 F/F ;LysM Cre mice starting from 4 days after left anterior descending (LAD) artery ligation compared with those in EP3 F/F controls ( Fig. 3b ), through suppression of recruitment of CD11b + Ly6G − CD115 + Ly6C low Mos/Mps ( Fig. 3c ) not CD11b + Ly6G − CD115 + Ly6C high Mos/Mps ( Fig. 3d ), which was further confirmed by using additional F4/80 marker ( Supplementary Fig. 4a–e ). While myeloid- Ep3 deficiency had no significant effect on total residential Mps in spleens, lungs, livers and hearts ( Supplementary Fig. 5a–d ), and on circulating Mos and neutrophils in mice either ( Supplementary Fig. 6a,b ). Again, Mo adoptive transfer confirmed Ep3 deficiency resulted in decreased Ly6C low infiltration without overt influence on Ly6C high differentiation in circulation and infracted hearts ( Supplementary Fig. 7a–i ). The Ly6C low Mo/Mp surface marker CX3CR1 and VEGF expression in the infiltrated Mos/Mps were reduced by half in Ep3 F/F ;LysM Cre mice ( Fig. 3e ), and the CX3CR1 ligand CX3CL1 expression was not altered in hearts from Ep3 F/F ;LysM Cre mice ( Supplementary Fig. 8a–c ). Moreover, Ep3 deletion did not influence proliferation and apoptosis of Mos/Mps infiltrated in infarcted hearts ( Supplementary Fig. 9a–d ). Immunostaining further confirmed reduction of VEGF expression in Mos/Mps in injured hearts in Ep3 F/F ;LysM Cre mice ( Fig. 3f,g ). Accordingly, in Ep3 F/F ;LysM Cre mice, neovascularization in the ischaemic zone at a late stage (day 14 after LAD ligation) was also diminished ( Fig. 3h–j ), infarct areas were expanded ( Supplementary Fig. 10a,b ), and cardiac function recovery was markedly impaired after MI ( Fig. 3k,l , Supplementary Fig. 10c , Supplementary Table 1 ). However, Ep3 F/F ;LysM Cre mice had normal cardiac function at basal condition and even after dobutamine challenge ( Supplementary Table 2 ), and Ep3 deficiency did not influence the number and functions of neutrophil infiltrated in the infarcted hearts ( Supplementary Fig. 11a–h ). 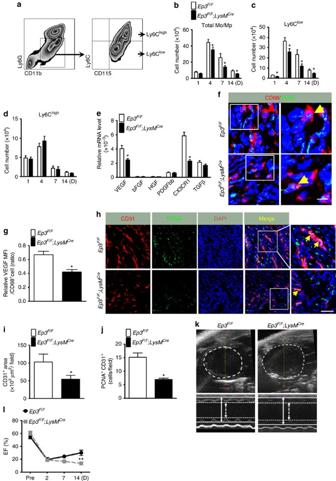Figure 3:Ep3deletion retards cardiac recovery after MI in mice. (a) Gating strategy for CD11b+CD115+Ly6G−Ly6Chighand CD11b+CD115+Ly6G−Ly6ClowMos/Mps in hearts after left anterior descending (LAD) artery ligation in mice. (b–d) Effect ofEp3deletion on recruitment of total Mos/Mps (b), Ly6Clow(c) and Ly6Chigh(d) Mos/Mps in injured hearts of mice after MI. Data represent mean±s.e.m. *P<0.05 versusEp3F/F(unpaired two-tailedt-test);n=5–8. (e) mRNA expression levels ofVEGF, fibrolast growth factor (FGF), hepatocyte growth factor (HGF), platelet-derived growth factor-bb (PDGFbb), andCX3CR1in Mos/Mps sorted from hearts inEp3F/FandEp3F/F;LysMCremice at day 14 post MI. Data represent mean±s.e.m. *P<0.05 versusEp3F/F(unpaired two-tailedt-test);n=10. (f) Representative immunostaining for CD68 (red) and VEGF (green) in peri-infarct zones of hearts fromEp3F/FandEp3F/F;LysMCremice at day 14 post MI. The solid box outlines the region enlarged to the right. Yellow arrow, CD68+/VEGF+cell. Scale bar, 5 μm. (g) Quantitation of VEGF signalling in CD68+cells in injured hearts as shown inf. Data represent mean±s.e.m. *P<0.05 versusEp3F/F(unpaired two-tailedt-test);n=5. (h) Representative immunostaining of CD31 (red) and proliferating cell nuclear antigen (PCNA, green) in peri-infarct zones of hearts fromEp3F/FandEp3F/F;LysMCremice at day 14 post MI. The solid box outlines the region enlarged to the right; yellow arrow, CD31+/PCNA+cell. Scale bar, 20 μm. (i,j) Quantitation of CD31+areas (i) and PCNA+CD31+cells (j) in injured hearts as shown inh. Data represent mean±s.e.m. *P<0.05 versusEp3F/F(unpaired two-tailedt-test);n=7. (k) Representative echocardiography images with M-mode views of infarcted hearts fromEp3F/F;LysMCreandEp3F/Fmice on day 14 after MI. Arrows and lines mark left ventricular inner diameters (LVID) in systole (dashed) and diastole (firm). (l) Cardiac function ofEp3F/F;LysMCreandEp3F/Fmice at different timepoints after MI. EF, ejection fraction. *P<0.05 versusEp3F/F(unpaired two-tailedt-test);n=9–13. Figure 3: Ep3 deletion retards cardiac recovery after MI in mice. ( a ) Gating strategy for CD11b + CD115 + Ly6G − Ly6C high and CD11b + CD115 + Ly6G − Ly6C low Mos/Mps in hearts after left anterior descending (LAD) artery ligation in mice. ( b – d ) Effect of Ep3 deletion on recruitment of total Mos/Mps ( b ), Ly6C low ( c ) and Ly6C high ( d ) Mos/Mps in injured hearts of mice after MI. Data represent mean±s.e.m. * P <0.05 versus Ep3 F/F (unpaired two-tailed t -test); n =5–8. ( e ) mRNA expression levels of VEGF , fibrolast growth factor ( FGF ), hepatocyte growth factor ( HGF ), platelet-derived growth factor-bb ( PDGFbb ), and CX3CR1 in Mos/Mps sorted from hearts in Ep3 F/F and Ep3 F/F ;LysM Cre mice at day 14 post MI. Data represent mean±s.e.m. * P <0.05 versus Ep3 F/F (unpaired two-tailed t -test); n =10. ( f ) Representative immunostaining for CD68 (red) and VEGF (green) in peri-infarct zones of hearts from Ep3 F/F and Ep3 F/F ;LysM Cre mice at day 14 post MI. The solid box outlines the region enlarged to the right. Yellow arrow, CD68 + /VEGF + cell. Scale bar, 5 μm. ( g ) Quantitation of VEGF signalling in CD68 + cells in injured hearts as shown in f . Data represent mean±s.e.m. * P <0.05 versus Ep3 F/F (unpaired two-tailed t -test); n =5. ( h ) Representative immunostaining of CD31 (red) and proliferating cell nuclear antigen (PCNA, green) in peri-infarct zones of hearts from Ep3 F/F and Ep3 F/F ;LysM Cre mice at day 14 post MI. The solid box outlines the region enlarged to the right; yellow arrow, CD31 + /PCNA + cell. Scale bar, 20 μm. ( i , j ) Quantitation of CD31 + areas ( i ) and PCNA + CD31 + cells ( j ) in injured hearts as shown in h . Data represent mean±s.e.m. * P <0.05 versus Ep3 F/F (unpaired two-tailed t -test); n =7. ( k ) Representative echocardiography images with M-mode views of infarcted hearts from Ep3 F/F ;LysM Cre and Ep3 F/F mice on day 14 after MI. Arrows and lines mark left ventricular inner diameters (LVID) in systole (dashed) and diastole (firm). ( l ) Cardiac function of Ep3 F/F ;LysM Cre and Ep3 F/F mice at different timepoints after MI. EF, ejection fraction. * P <0.05 versus Ep3 F/F (unpaired two-tailed t -test); n =9–13. Full size image Mps, as the major source of matrix metallopeptidases (MMPs) and TGFβ1, play an important role in cardiac remodelling and fibrosis [18] . Mo/Mp-Ep3 deletion, indeed, caused less non-vascular smooth muscle actin (SMA) positive myofibroblasts ( Supplementary Fig. 12a,b ), downregulation of MMP9 , collagen I, III and Thrombospondin1 ( THBS1 ) expression in infarcted hearts in mice ( Supplementary Fig. 12c–j ). Consistently, Masson’s trichrome staining showed an increased myocardial scar size with decreased collagen deposition in Ep3 F/F ;LysM Cre mice at both day 7 and 14 after MI ( Supplementary Fig. 13a–c ). We did not observe significant difference of early necrotic area between Ep3 F/F ;LysM Cre and Ep3 F/F mice after MI ( Supplementary Fig. 13d,e ). Taken together, myeloid-Ep3 deletion impairs cardiac recovery from infarction by suppression of Ly6C low Mo/Mp-mediated angiogenesis and cardiac fibrosis in mice ( Supplementary Table 3 ). Given that Ep3 deficiency inhibited VEGF expression in reparative Ly6C low Mps, we tested the effect of the Mp Ep3 receptor on angiogenesis in vitro . Indeed, VEGF expression was diminished at both the mRNA ( Supplementary Fig. 14a ) and protein levels ( Supplementary Fig. 14b,c ) in cultured Mps from Ep3 F/F ;LysM Cre mice. In a cultured three-dimensional angiogenesis model using HUVECs, their sprouting and tube structure formations were markedly reduced when co-cultured with peritoneal Mps from Ep3 F/F ;LysM Cre mice compared to those in models co-cultured from Ep3 F/F controls ( Supplementary Fig. 14d–g ). To validate the role of Ep3 receptor in Mos/Mps, we examined whether bone marrow transplantation (BMT) from wild-type (WT) donors could rescue the defective function of Ly6C low Mos/Mps in Ep3 knockout (KO) mice. Genotyping of both tail specimens and blood samples verified successful BM reconstitution ( Fig. 4a ). Notably, total Ly6C low , not Ly6C high Mos/Mps recruited in ischaemic hearts were significantly reduced in WT mice which underwent BMT from Ep3 KO mice BM (KO→WT) ( Fig. 4b–d ). Moreover, the decreased expression of both VEGF and CX3CR1 in EP3 KO Ly6C low Mos/Mps in the infarcted hearts was completely rectified by WT BMT (WT→KO, Fig. 4e ). In line with the recovered infiltration and function of Ly6C low Mos/Mps, neovascularization in peri-infarct zones and cardiac function after MI were significantly improved in WT→KO mice as compared with that in KO→KO mice ( Fig. 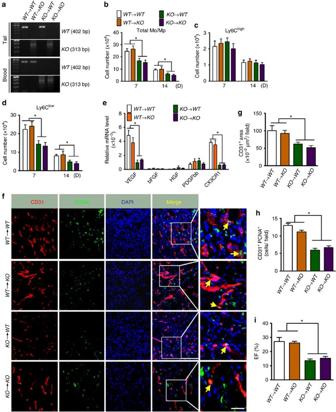Figure 4: BMT ameliorates impaired cardiac function after MI in EP3 KO mice. (a) Bone marrow transplantation (BMT) betweenEp3KO and WT mice was confirmed by genotyping. (b–d) Recruitment of total Mos/Mps (b), Ly6Chigh(c) and Ly6Clow(d) Mos/Mps in injured hearts in chimeric mice that underwent BMT. Data represent mean±s.e.m. *P<0.05 as indicated (unpaired two-tailedt-test);n=6–7. (e) mRNA expression levels ofVEGF, FGF, HGF, PDGFbbandCX3CR1in Mos/Mps sorted from hearts from BMT chimeric mice at day 14 post MI. Data represent mean±s.e.m. *P<0.05 as indicated (unpaired two-tailedt-test);n=4. (f) Representative immunostaining of CD31 (red) and PCNA (green) in peri-infarct zones of hearts from BMT chimeric mice at day 14 post MI. The solid box outlines the region enlarged to the right. Yellow arrow, CD31+/PCNA+cells. Scale bar, 20 μm. (g,h) Quantitation of CD31+areas (g) and PCNA+CD31+cells (h) in injured hearts as shown inf. Data represent mean±s.e.m. *P<0.05 as indicated (unpaired two-tailedt-test);n=6–7. (i) Cardiac function of BMT chimeric mice at day 14 after MI. EF, ejection fraction. Data represent mean±s.e.m. *P<0.05 as indicated (unpaired two-tailedt-test);n=8–11. 4f–i , Supplementary Table 4 ). Figure 4: BMT ameliorates impaired cardiac function after MI in EP3 KO mice. ( a ) Bone marrow transplantation (BMT) between Ep3 KO and WT mice was confirmed by genotyping. ( b – d ) Recruitment of total Mos/Mps ( b ), Ly6C high ( c ) and Ly6C low ( d ) Mos/Mps in injured hearts in chimeric mice that underwent BMT. Data represent mean±s.e.m. * P <0.05 as indicated (unpaired two-tailed t -test); n =6–7. ( e ) mRNA expression levels of VEGF, FGF, HGF, PDGFbb and CX3CR1 in Mos/Mps sorted from hearts from BMT chimeric mice at day 14 post MI. Data represent mean±s.e.m. * P <0.05 as indicated (unpaired two-tailed t -test); n =4. ( f ) Representative immunostaining of CD31 (red) and PCNA (green) in peri-infarct zones of hearts from BMT chimeric mice at day 14 post MI. The solid box outlines the region enlarged to the right. Yellow arrow, CD31 + /PCNA + cells. Scale bar, 20 μm. ( g , h ) Quantitation of CD31 + areas ( g ) and PCNA + CD31 + cells ( h ) in injured hearts as shown in f . Data represent mean±s.e.m. * P <0.05 as indicated (unpaired two-tailed t- test); n =6–7. ( i ) Cardiac function of BMT chimeric mice at day 14 after MI. EF, ejection fraction. Data represent mean±s.e.m. * P <0.05 as indicated (unpaired two-tailed t -test); n =8–11. Full size image Ep3 deficiency inhibits CX3CR1 and VEGF expression in Mps Reparative Ly6C low Mo/Mp recruitment during inflammation, including that post MI, depends on the CX3CR1 receptor [6] . We detected striking downregulation of CX3CR1 and VEGF expression in peritoneal Mps isolated from Ep3 F/F ;LysM Cre mice challenged by zymosan at both 48 h ( Fig. 5a , Supplementary Fig. 15a ) and 96 h ( Fig. 5b , Supplementary Fig. 15b ) and in cultured Ep3 -deficient Mps ( Ep3 F/F ;LysM Cre mice) treated by PGE 2 ( Fig. 5c , Supplementary Fig. 15c ). CCR2, the receptor for monocyte chemoattractant protein-1 (MCP-1) that mediates pro-inflammatory Ly6C high Mo/Mp recruitment, was not altered significantly in Ep3 -deficient Mps ( Fig. 5a–c ). Accordingly, the migration of Ep3 -deficient Mps in Boyden chambers was notably restrained in Ep3 -deficient Mps with and without PGE 2 stimulation ( Fig. 5d ). 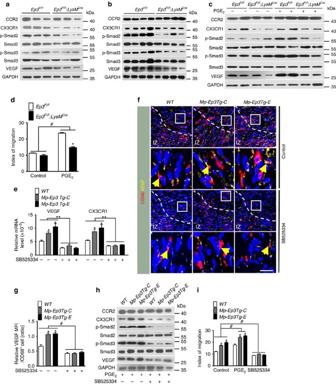Figure 5:Ep3regulates CX3CR1 and VEGF expression through TGFβ1 signalling. (a,b)Western blot analysis of CCR2, CX3CR1, phospho-Smad2, phospho-Smad3 and VEGF in Mos/Mps fromEp3F/FandEp3F/F;LysMCremice at 16 h (a) and 96 h (b)after a zymosan challenge. (c) Western blot analysis of CCR2, CX3CR1, phospho-Smad2, phospho-Smad3 and VEGF in cultured Mps with or without PGE2stimulation. (d) Effect ofEp3deletion on Mp migration in response to PGE2. Data represent mean±s.e.m. *P<0.05 versusEp3F/F,#P<0.05 as indicated (unpaired two-tailedt-test);n=5. (e) Effect of TGFβ1 blocker SB525334 on Ep3-mediatedVEGFandCX3CR1mRNA expression in cultured Mps.Mp-Ep3Tg, Mp-specificEp3αtransgenic mice. Data represent mean±s.e.m. *P<0.05 versus wild-type (WT), **P<0.01 versus indicated (unpaired two-tailedt-test);n=5. (f) Representative immunostaining of CD68 (red) and VEGF (green) in peri-infarct zones of hearts fromMp-Ep3Tgmice at day 14 post MI. The solid box outlines the region enlarged below. Yellow arrow, CD68+/VEGF+cells. Scale bar 20 μm. IZ, infarct zone. (g) Quantitation of VEGF signalling in CD68+cells in injured hearts as shown inf. Data represent mean±s.e.m. *P<0.05 versus WT,#P<0.05 as indicated (unpaired two-tailedt-test);n=5. (h) Effect of SB525334 onEp3-mediated VEGF and CX3CR1 protein expression in cultured Mps. (i) Effect of SB525334 on PGE2/Ep3-mediated Mp migrationin vitro. Data represent mean±s.e.m. *P<0.05 versus WT,#P<0.05 as indicated (unpaired two-tailedt-test);n=4–6. Figure 5: Ep3 regulates CX3CR1 and VEGF expression through TGFβ1 signalling. ( a , b )Western blot analysis of CCR2, CX3CR1, phospho-Smad2, phospho-Smad3 and VEGF in Mos/Mps from Ep3 F/F and Ep3 F/F ;LysM Cre mice at 16 h ( a ) and 96 h ( b )after a zymosan challenge. ( c ) Western blot analysis of CCR2, CX3CR1, phospho-Smad2, phospho-Smad3 and VEGF in cultured Mps with or without PGE 2 stimulation. ( d ) Effect of Ep3 deletion on Mp migration in response to PGE 2 . Data represent mean±s.e.m. * P <0.05 versus Ep3 F/F , # P <0.05 as indicated (unpaired two-tailed t -test); n =5. ( e ) Effect of TGFβ1 blocker SB525334 on Ep3-mediated VEGF and CX3CR1 mRNA expression in cultured Mps. Mp-Ep3Tg , Mp-specific Ep3α transgenic mice. Data represent mean±s.e.m. * P <0.05 versus wild-type (WT), ** P <0.01 versus indicated (unpaired two-tailed t -test); n =5. ( f ) Representative immunostaining of CD68 (red) and VEGF (green) in peri-infarct zones of hearts from Mp-Ep3Tg mice at day 14 post MI. The solid box outlines the region enlarged below. Yellow arrow, CD68 + /VEGF + cells. Scale bar 20 μm. IZ, infarct zone. ( g ) Quantitation of VEGF signalling in CD68 + cells in injured hearts as shown in f . Data represent mean±s.e.m. * P <0.05 versus WT, # P <0.05 as indicated (unpaired two-tailed t -test); n =5. ( h ) Effect of SB525334 on Ep3 -mediated VEGF and CX3CR1 protein expression in cultured Mps. ( i ) Effect of SB525334 on PGE 2 / Ep3 -mediated Mp migration in vitro . Data represent mean±s.e.m. * P <0.05 versus WT, # P <0.05 as indicated (unpaired two-tailed t -test); n =4–6. Full size image Previously, we demonstrated that the Ep3 receptor mediates TGFβ1 signalling in pulmonary vascular smooth muscle cells by activation of Rho/ROCK [19] . Similarly, TGFβ1 signalling (phosphorylation of Smad2 and Smad3) was inhibited in Ep3 -deficient Mps both in vivo and in vitro ( Fig. 5a–c , Supplementary Fig. 15a–c ). Additionally, Ep3 deletion suppressed mouse Mp migration in response to PGE 2 ( Fig. 5d ). In human blood CD14 dim CD16 + Mos are similar to reparative Ly6C low mouse Mos (ref. 20 ). Ep3 agonist sulprostone promoted the migration of human CD14 dim CD16 + Mos, while Ep3 inhibitor L798106 suppressed CD14 dim CD16 + Mo migration ( Supplementary Fig. 16a,b ). Likewise, Ep3 receptor was also involved in regulation of CX3CR1 expression in human Mos ( Supplementary Fig. 16c ). To investigate whether TGFβ1 signalling is involved in Ep3 -mediated regulation of CX3CR1 and VEGF expression in Mos/Mps, we created an Mp-specific Ep3α transgenic (Mp-EP3Tg) mouse model using the CD68 promoter ( Supplementary Fig. 17a–d ). Indeed, overexpression of Mp-Ep3α induced activation of TGFβ1 signalling and elevated expression of both VEGF and CX3CR1 in Mps ( Fig. 5e–h , Supplementary Fig. 18 ), and therefore increased PGE 2 -induced Mp migration ( Fig. 5i ), promoted infiltration of Ly6C low Mos/Mps ( Fig. 6a–c ) and angiogenesis ( Fig. 6d–f ) in the infarcts, and facilitated cardiac recovery after MI ( Fig. 6g ). Interestingly, inhibition of TGFβ1 signalling markedly diminished the induction of VEGF and CX3CR1 expression ( Fig. 5e–h ) and augmented migration capacity in vitro in Ep3α -overexpressed Mps ( Fig. 5i ), retarded the increased Ly6C low Mos/Mps accumulation in infarcts ( Fig. 6c ), and enhanced neovascularization in peri-infarct zones and cardiac function in Mp-Ep3αTg mice ( Fig. 6d–g , Supplementary Table 5 ). We then tested whether the TGFβ1 pathway is implicated in Mp-Ep3 -mediated angiogenesis using an Mp/HUVEC co-culture system. As shown in Supplementary Fig. 19a–c , forced expression of Ep3α in Mps increased VEGF expression at both the mRNA and protein levels, while the TGFβ1 signalling blocker SB525334 attenuated the elevated VEGF expression in Mp-Ep3Tg mice. Moreover, more sprouts and tubal structures from HUVECs containing beads were formed in culture with Mps from Mp-Ep3Tg mice than with those from WT controls ( Supplementary Fig. 19d–g ). Again, these differences were lost by the addition of SB525334 ( Supplementary Fig. 19d–g ). Thus, Ep3 -mediated reparative Ly6C low Mo/Mp recruitment and neovascularization in infarcted hearts is dependent on TGFβ1 signalling. 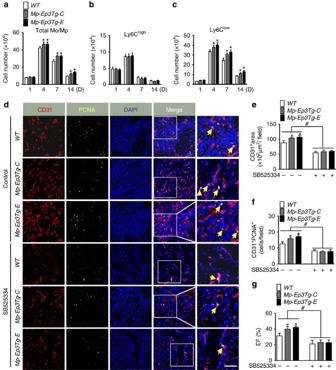Figure 6:Ep3overexpression in Mos/Mps improves cardiac recovery after MI in mice. (a–c) Effect ofEp3 overexpression on recruitment of total Mos/Mps (c), Ly6Chigh, (d) and Ly6ClowMos/Mps in injured hearts mice after MI. Data represent mean±s.e.m. *P<0.05 versus WT (unpaired two-tailedt-test);n=5–7. (d) Representative immunostainings of CD31 (red) and PCNA (yellow) in peri-infarct zones of hearts fromWT, Mp-Ep3Tg-CandMp-Ep3Tg-Emice at day 14 post-MI. The solid box outlines the region enlarged to the right; yellow arrow, CD31+/PCNA+cell. Scale bar, 20 μm. (e,f) Quantitation of CD31+areas (e) and PCNA+CD31+cells (f) in injured hearts, as shown ind. Data represent mean±s.e.m. *P<0.05 versus WT,#P<0.05 as indicated(unpaired two-tailedt-test);n=6. (g) Cardiac function ofWT, Mp-Ep3Tg-CandMp-Ep3Tg-Emice at day 14 after MI. Data represent mean±s.e.m. *P<0.05 versus WT,#P<0.05 as indicated (unpaired two-tailedt-test);n=7–8. Figure 6: Ep3 overexpression in Mos/Mps improves cardiac recovery after MI in mice. ( a – c ) Effect of Ep3 o verexpression on recruitment of total Mos/Mps ( c ), Ly6C high , ( d ) and Ly6C low Mos/Mps in injured hearts mice after MI. Data represent mean±s.e.m. * P <0.05 versus WT (unpaired two-tailed t -test); n =5–7. ( d ) Representative immunostainings of CD31 (red) and PCNA (yellow) in peri-infarct zones of hearts from WT, Mp-Ep3Tg-C and Mp-Ep3Tg-E mice at day 14 post-MI. The solid box outlines the region enlarged to the right; yellow arrow, CD31 + /PCNA + cell. Scale bar, 20 μm. ( e , f ) Quantitation of CD31 + areas ( e ) and PCNA + CD31 + cells ( f ) in injured hearts, as shown in d . Data represent mean±s.e.m. * P <0.05 versus WT, # P <0.05 as indicated(unpaired two-tailed t -test); n =6. ( g ) Cardiac function of WT, Mp-Ep3Tg-C and Mp-Ep3Tg-E mice at day 14 after MI. Data represent mean±s.e.m. * P <0.05 versus WT, # P <0.05 as indicated (unpaired two-tailed t -test); n =7–8. Full size image CX3CR1 and VEGF are downstream targets of TGFβ1 Through the PWMScan tool, 4 and 2 potential Smad binding elements (SBEs) were predicted in the promoter of murine Cx3cr1 (S1–4) and Vegf (S1′–2′) genes, respectively ( Fig. 7a,b ). However, the fragments containing S3 and S4 SBEs in the promoter of Cx3cr1 were detected in the anti-Smad2/3 immunocomplex by Chip assay in mouse RAW264.7 cell line ( Fig. 7c ). Activation of TGFβ1 signalling by co-transfection of the TGFβ receptor Alk5 or addition of exogenous TGFβ1 markedly enhanced luciferase activities in the Cx3cr1 promoter (S3+S4) containing reporter-transfected RAW264.7 cells, both of which could be specifically blocked by a TGFβ1 inhibitor ( Fig. 7d ). Mutation of either S3 or S4 significantly weakened the TGFβ1 and Alk5 co-transfection-induced luciferase activities in RAW264.7 cells as compared to these of WT fragment (S3+S4) transfected cells ( Fig. 7e ). Moreover, Ep3 inhibition also suppressed S3+S4 promoter-driven activity in a dose-dependent manner ( Fig. 7f ). Similarly, two SBEs (S1′ and S2′) were identified in the VEGF promoter region by Chip and luciferase assays ( Fig. 7g–i ) in RAW264.7 cells. Moreover, 1 and 5 potential SBEs were predicted in the promoter of human CX3CR1 (hS) and VEGF genes (hS1′–hS5′, Fig. 7j,k ), respectively. Using a human THP-1 cell line, we identified one (hS, Fig. 7l–n ) and three (hS3′–hS5′, Fig. 7o–q ) functional SBEs in promoter of human CX3CR1 and VEGF genes, respectively. Therefore, activation of the EP3 receptor induces CX3CR1 and VEGF expression in Mps through TGFβ1 signalling and subsequently promotes Ly6C low accumulation after MI and peri-infarct angiogenesis ( Fig. 7r ). 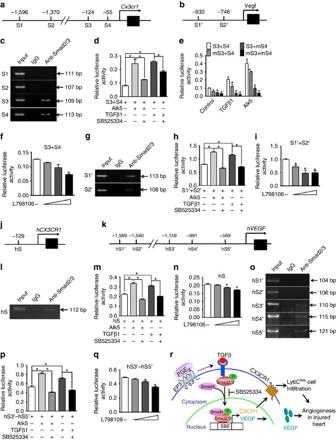Figure 7: CX3CR1 and VEGF are TGFβ1-targeting genes in mice and humans. (a,b) Schematic illustration of predicted Smad binding elements (SBEs) in the promoter of murineCx3cr1(a) andVegf(b) genes. S=SBE. (c) Gel electrophoresis of PCR-amplified SBE-containing fragments in the promoter of the murineCx3cr1gene using anti-Smad2/3 immunoprecipitation. (d) Effect of the TGFβ1 blocker SB525334 on S3+S4 fragment-mediated luciferase activity. *P<0.05 as indicated (unpaired two-tailedt-test);n=4. (e) Effect of mutations of S3 (mS3) and S4 (mS4) on S3+S4 fragment-mediated transcription activity. *P<0.05 versus the S3+S4 group,n=4. (f) Effect of L-798,106 on S3+S4 fragment-mediated luciferase activity in RAW264.7 cells. *P<0.05 versus no treatment (unpaired two-tailedt-test);n=4. (g) Gel electrophoresis of PCR-amplified SBE-containing fragments in the promoter of the murineVegfgene using anti-Smad2/3 immunoprecipitation. (h) Effect of SB525334 on the functional SBEs (S1′+S2′) in murineVegfpromoter. *P<0.05 as indicated (unpaired two-tailedt-test);n=4. (i) Effect of L798106 on S1′+S2′ fragment-mediated luciferase activity in RAW264.7 cells. *P<0.05 versus no treatment (unpaired two-tailedt-test);n=5. (j,k) Schematic illustration of the predicted SBE(s) on the humanCX3CR1gene (hS, (j)) and the humanVEGFgene (hS′, (k)). (l) Gel electrophoresis of PCR-amplified SBE-containing fragments in the promoter of the humanCX3CR1gene. (m) Effect of SB525334 on hS-mediated transcription activity in THP-1 cells. *P<0.05 as indicated (unpaired two-tailedt-test);n=5. (n) Effect of L-798,106 on hS-mediated transcription activity in THP-1 cells. *P<0.05 versus no treatment (unpaired two-tailedt-test);n=5. (o) Gel electrophoresis of PCR-amplified SBE-containing fragments in the promoter of the humanVEGFgene. (p) Effect of SB525334 on hS3′–hS5′ fragment-mediated transcription activity in THP-1 cells. *P<0.05 as indicated,n=5. (q) Effect of L-798,106 on hS3′–hS5′ fragment-mediated transcription activity in THP-1 cells. *P<0.05 versus no treatment (unpaired two-tailedt-test);n=5. (r) Schematic diagram of EP3-mediated regulation of CX3CR1 and VEGF genes in Mos/Mps through TGFβ1. Figure 7: CX3CR1 and VEGF are TGFβ1-targeting genes in mice and humans. ( a , b ) Schematic illustration of predicted Smad binding elements (SBEs) in the promoter of murine Cx3cr1 ( a ) and Vegf ( b ) genes. S=SBE. ( c ) Gel electrophoresis of PCR-amplified SBE-containing fragments in the promoter of the murine Cx3cr1 gene using anti-Smad2/3 immunoprecipitation. ( d ) Effect of the TGFβ1 blocker SB525334 on S3+S4 fragment-mediated luciferase activity. * P <0.05 as indicated (unpaired two-tailed t -test); n =4. ( e ) Effect of mutations of S3 (mS3) and S4 (mS4) on S3+S4 fragment-mediated transcription activity. * P <0.05 versus the S3+S4 group, n =4. ( f ) Effect of L-798,106 on S3+S4 fragment-mediated luciferase activity in RAW264.7 cells. * P <0.05 versus no treatment (unpaired two-tailed t -test); n =4. ( g ) Gel electrophoresis of PCR-amplified SBE-containing fragments in the promoter of the murine Vegf gene using anti-Smad2/3 immunoprecipitation. ( h ) Effect of SB525334 on the functional SBEs (S1′+S2′) in murine Vegf promoter. * P <0.05 as indicated (unpaired two-tailed t -test); n =4. ( i ) Effect of L798106 on S1′+S2′ fragment-mediated luciferase activity in RAW264.7 cells. * P <0.05 versus no treatment (unpaired two-tailed t -test); n =5. ( j , k ) Schematic illustration of the predicted SBE(s) on the human CX3CR1 gene (hS, ( j )) and the human VEGF gene (hS′, ( k )). ( l ) Gel electrophoresis of PCR-amplified SBE-containing fragments in the promoter of the human CX3CR1 gene. ( m ) Effect of SB525334 on hS-mediated transcription activity in THP-1 cells. * P <0.05 as indicated (unpaired two-tailed t -test); n =5. ( n ) Effect of L-798,106 on hS-mediated transcription activity in THP-1 cells. * P <0.05 versus no treatment (unpaired two-tailed t -test); n =5. ( o ) Gel electrophoresis of PCR-amplified SBE-containing fragments in the promoter of the human VEGF gene. ( p ) Effect of SB525334 on hS3′–hS5′ fragment-mediated transcription activity in THP-1 cells. * P <0.05 as indicated, n =5. ( q ) Effect of L-798,106 on hS3′–hS5′ fragment-mediated transcription activity in THP-1 cells. * P <0.05 versus no treatment (unpaired two-tailed t -test); n =5. ( r ) Schematic diagram of EP3-mediated regulation of CX3CR1 and VEGF genes in Mos/Mps through TGFβ1. Full size image PGE 2 is implicated in the regulation of multiple aspects of inflammation by tuning the functions of different immune cells, including Mos/Mps [21] . Mos/Mps are a dominant source of PGE 2 at sites of inflammation [22] . In mice, Mos/Mps can be divided into two subsets based on the expression level of Ly6C (pro-inflammatory Ly6C high and less inflammatory and patrolling Ly6C low ) [6] . In humans, CD14 + CD16 − Mos are similar to murine Ly6C high cells, while CD14 dim Mos are similar to murine Ly6C low Mos [20] . We found that Ep3 mediates recruitment and reparative function of Ly6C low Mo/Mp in inflamed tissues. Activation of the Ep3 receptor upregulates expression of the Mp chemokine receptor CX3CR1, which mediates Ly6C low Mo infiltration in hearts after MI [6] . In addition, the Mo/Mp Ep3 receptor also mediates expression of the pro-angiogenic factor VEGF, which stimulates wound healing after MI by enhancing neovascularization in peri-infarct zones in mice. In agreement with our observations, tumour-derived PGE 2 promotes differentiation of tumour-associated suppressive Mps (M2-like Mps) from the Mos infiltrated in tumours [23] . And the PGE 2 – Ep3 axis also mediates recruitment and maturation of mast cells upon repeated allergen challenges [24] . The Ep3 receptor mediates multiple cellular cascades by activating different types of heterotrimeric G proteins, including Gαs, Gαi and Gα12/13 (refs 25 , 26 ). We recently discovered that activation of the Ep3 receptor augments Rho/ROCK-dependent TGFβ1/Smad2/3 signalling to facilitate hypoxia-induced vascular fibrosis by coupling with Gα12 in pulmonary arterial smooth muscle cells [19] . Indeed, Ep3 deficiency also results in decreased Rho activity and subsequent suppression of TGFβ1 signalling in both peritoneal and infarcted myocardium-derived Mps, whereas forced expression of the Ep3 receptor in Mos/Mps amplified TGFβ1/Smad2/3 signalling. Furthermore, we identified conservative SBEs in the promoter regions of both human and mouse CX3CR1 genes coding a chemokine receptor for CX3CL1 , which governs Ly6C low Mo migration into inflammation sites [6] . Thus, the Ep3 receptor regulates Ly6C low Mo/Mp recruitment into the ischaemic myocardium through the TGFβ1/CX3CR1 pathway. Interestingly, CX3CR1/CX3CL1 interactions confer a vital survival signal for Mos/Mps, whose complete disruption causes death of peripheral Mos [27] and renal resident Mps [28] , [29] and forms cells in atherosclerosis plaques [27] . We failed to observe marked death and/or apoptosis of peripheral Mos or Mps in the injured myocardium in Mp- Ep3-deficient mice with reduced expression of CX3CR1 in Mos/Mps, which is consistent with the phenotypes presented in CX3CR1 heterozygous mice ( CX3CR1 GFP/+ ) [27] , [30] . In addition, CX3CR1 deficiency appears to impair reparative functions of macrophages (pro-fibrosis, proangiogenesis, and phagocytosis) in a variety of disease processes, such as skin wound healing [31] , [32] , [33] . In an experimental MI mouse model, Mo/Mp Ep3 deletion retarded myocardial healing by inhibiting peri-infarct angiogenesis. Further mechanistic analysis revealed that Ep3 receptor activation in Mos/Mps promotes TGFβ1/Smad pathway-derived VEGF transcription. As previously reported [34] , we validated multiple conservative SBEs in the VEGF gene promoter in both mouse and human Mp cell lines, but not in infiltrated cardiac Mo/Mps due to technical difficulties. Taken together, the data suggest that activation of the Mo/Mp Ep3 receptor facilitates wound healing after MI by increasing CX3CR1-mediated Ly6C low Mo recruitment and VEGF-induced angiogenesis, which are TGFβ1/Smad pathway-dependent. Cardiac PGE 2 generation increases during acute MI [17] . Despite the expression of multiple PGE 2 receptor subtypes in hearts, selective stimulation of the Ep3 receptor displays cardio-protection against ischaemia/reperfusion injury in different mammalian species [35] , [36] , [37] , [38] . For instance, pharmacological activation of Ep3 receptor reduces myocardial infarct size in rodents by activation of protein kinase C (PKC) and the opening of ATP-sensitive potassium channels in cardiomyocytes [36] , [37] . We found that inactivation of Ep3 in Mos/Mps impairs myocardial repair after acute ischaemia; in contrast, forced activation of Ep3 -mediated signalling in Mos/Mps accelerates healing in mice after MI by increasing recruitment of reparative Mos/Mps and secretion of proangiogenic VEGF. Thus, Ep3 mediates cardiac protection against ischaemia, at least in part through activation of reparative Mos/Mps. In addition, Ep3 is also involved in regulation of lipid metabolism. Global Ep3 deletion promotes to diet-induced obesity and exaggerates ectopic lipid deposition such as in skeletal muscle in mice [39] , [40] . Hepatic Ep3 deficiency exacerbated atherosclerosis in hyperlidemic mice through suppression of biliary cholesterol secretion in mice [41] . However, Ep3 mediates vasoconstriction [42] , and genetic deletion of Ep3 receptor increases bleeding tendency [38] and reduces atherosclerosis-related thrombosis [43] , suggesting Ep3 involvement in platelet activation. Therefore, the potential efficacy of specific activation of Ep3 receptor in cardiac recovery after MI requires further investigations. In summary, we showed that the PGE 2 – Ep3 axis in Mo/Mp exerts a beneficial effect on myocardial recovery in response to acute ischaemia through TGFβ1-mediated activation of reparative Ly6C low Mos/Mps. These observations suggest Ep3 receptor and its downstream pathway maybe a promising therapeutic target for acute MI. Mice All animal procedures were approved by the Institutional Animal Care and Use Committee of the Institute for Nutritional Sciences, Chinese Academy of Sciences, as well as the number of animals to be used were approved based on the expected effects size. Ep3 F/F ( Ep3 F/F ) [44] and Ep3 knockout (KO) mice [19] were maintained on C57BL/6 background, LysM Cre transgenic mice (C57BL/6, The Jackson Laboratory) were crossed Ep3 F/F to obtain Ep3 F/F ;LysM Cre mice. Echocardiography High-resolution echocardiography imaging system (Vevo 770, Visual Sonics) were used with M-mode analysis to assess mouse cardiac function. Both male and female mice (10–14 weeks old) were anaesthetized by isoflurane inhalation (1–2%) and heart rate was maintained at 350–500 b.p.m. The mitral valve leaflet was visualized and cardiac function was evaluated in the parasternal long axis view as previously described [45] . Macrophage-specific Ep3α transgenic mice Macrophage (Mp)-specific Ep3α transgenic mice were generated as described previously [46] . Briefly, Ep3 α cDNA was cloned into the CD68 promoter-contained vector, and the successful construct was injected into C57BL6 zygotes to obtain founder mice. Mouse model of myocardial infarction Left anterior descending (LAD) ligation was used in both male and female mice (8–12 weeks old) to induce MI. Briefly, mice were anesthetized with isoflurane (2%) using an induction chamber, and the LAD coronary artery was completely ligated to induce left ventricular ischaemia [47] . Myocardial necrotic injury was assessed by nitro blue tetrazolium (NBT) staining as previously reported [48] . Briefly, hearts were collected 12 or 24 h after LAD ligation and then cut into slices about 2 mm thick. Slices were incubated in 0.5 mg ml −1 NBT in phosphate buffer at pH 7.4 and 37 °C for 20 min. The unstainedportion (necrotic) could be separated from the dark blue stained (non-necrotic) region. The percentage of necrotic area was determined by dividing the weight of the necrotic tissue by the total weight and multiplying by 100. As for infarction analysis, hearts were dissected at day 14 after infusion of 10% evans blue (100 μl) and frozen at −20 °C for 30 min, then cut into 2-mm-thick slices from apex to base. The slices were incubated in 1% triphenyltetrazolium chloride at 37 °C for 30 min to identify non-infarcted and infarcted areas. The normal myocardium was then recognized by red staining by triphenyltetrazolium chloride, while infarcted tissue presented as milky white. Infarct area was calculated as the ratio of the infarct area to the total slice areas previously described [49] . Enzyme-linked immunosorbent assay Serum was collected from retro-orbital blood from mice 14 days after MI induction. Levels of the heart failure marker brain natriuretic protein in serum was measured by enzyme-linked immunosorbent assay, according to the manufacturer’s instructions (R&D Systems). Immunofluorescence staining For immunofluorescence, heart sections (8 μm) were incubated with primary antibodies against CD68 (Serotec, 1:200), CD301 (Biolegend, 1:200), PCNA (CST, 1:800), CD31 (RD, 1:200), VEGF (Proteintech, 1:200), SMA (Sigma, 1:500), CollagenΙ(Proteintech,1:200), THBS1(Proteintech, 1:200) and Alexa Fluor 488/594/633-conjugated secondary antibodies (Invitrogen, Carlsbad, CA, 1:1,000) for 1 h at room temperature, respectively. The embedded hearts were washed and stained with DAPI (Millipore, MA). Images were captured under a Olympus (FV1000) laser-scanning confocal microscope from each heart section for further analysis. Positive staining area and relative mean fluorescent intensity were measured using Image-Pro Plus software 6.0 (Media Cybernetics, Rockville, MD, USA) [50] . For immunocytochemistry, primary Mos/Mps grown on slides were stimulated with or without PGE 2 and then fixed with 4% paraformaldehyde. The slides were blocked in TBST containing 1% bovine serum albumin after washing, incubated with primary antibodies against CD68 (Serotec, 1:200) or VEGF (Proteintech, 1:200) overnight at 4 °C, stained with a secondary antibody for 2 h at room temperature, and photographed using fluorescent microscopy as described above. At least five random images were taken in region of each slide and positive signalling was quantified as previously described [51] . Bone marrow transplantation Same sex BMT was performed as previously described [52] . In brief, mice (6–8 weeks old) were euthanized and bone marrow (BM) cells were collected from femurs and tibias. Recipient mice were lethally irradiated (one 5.0-Gy dose and another 4-Gy dose administered 1.5 h apart) from a 137Cs source (MDS Nordion, Ottawa, Ontario, Canada) and transplanted with 5 × 10 6 donor BM cells via tail vein injection to reconstitute the hematopoietic system. Eight weeks after transplantation, BMT chimeric mice were used for experiments. Fluorescence activated cell sorting analysis Cells collected from mice were stained with fluorochrome-conjugated antibodies, according to the manufacturer’s protocols. FITC-conjugated antibodies to CD11b (M1/70,1:50), Brilliant Violet 421-conjugated antibodies to CD115 (AFS98,1:50), APC-conjugated antibody to Ly6C (HK1.4,1:50), APC-CY7-conjugated antibody to Ly6G (1A8,1:50) were purchased from Biolegend. Flow cytometry was performed using a BD FACS Aria flow cytometry system (BD Biosciences, San Jose, CA), and data were analysed with FlowJo software. Total viable leukocyte number was determined with the trypan-blue exclusion method. Leukocyte subpopulation numbers were calculated as total leukocytes multiplied by per cent cells within the selected population gated by FlowJo software (Tree Star, Ashland, Ore) and all FACS gates for fluorochrome-labelled monoclonal antibodies were defined using appropriate isotype controls. Peritoneal inflammation Peritonitis was induced by intraperitoneal injection of zymosan (2 mg ml −1 ; Sigma-Aldrich, St Louis, MO). Peritoneal cells at different time points after the zymosan challenge were isolated for FACS analysis. Cell extract and culture Primary Mos/Mps were prepared from the abdominal cavity and cultured in 10% FBS 1640 medium. A single-cell suspension from infracted hearts was prepared as previously described [53] . Briefly, the hearts were dissected, carefully cut into small pieces with fine scissors, and enzymatically digested with 450 U ml −1 of a cocktail of type I collagenase, 125 U ml −1 type IX collagenase, and 60 U ml −1 DNase I, and 60 U ml −1 hyaluronidase I-S (Sigma, St Louis, MO) for 1 h at 37 °C. After digestion, the tissues were passed through 70-μm cell strainers, washed, and stained with antibody for FACS analysis. Western blot Cells were extracted in lysis buffer containing protease inhibitors. Protein concentration was determined by the BCA method using the Pierce BCA Protein Assay Kit (Pierce, Rockford, IL). Equal quantities of proteins from total cell lysates were separated by 10% SDS–PAGE gel and probed with antibodies against CX3CR1 (1:500, Abcam), CCR2 (1:500, Abcam), p-Smad2 (1:1,000, CST), p-Smad3 (1:1,000, CST), T-Smad3 (1:1,000, CST), T-Smad2/3 (1:1,000, CST), VEGF (1:1,000, Proteinteh), and GAPDH (1:2,000, CST), and then conjugated with an HRP-labelled secondary antibody in blocking buffer for 1–2 h at room temperature. Proteins were detected using an ECL detection kit (Super Signal West Pico Chemiluminescent Substrate), and signalling was quantified by image J software and presented as normalized arbitrary units. The uncropped scans of all western blots are supplied in Supplementary Fig. 20 . Macrophage (Mp) migration assay Primary Mps (1000,000 cells per well) were pretreated with 10 nM PGE 2 in serum-free DMEM media for 24 h and then seeded on cell culture inserts (Millicell-PCF, Millipore) with porous polycarbonate filters (8-μm pore size) in 24-well plates. DMEM with CX3CL1 (20 ng ml −1 ) was placed in the lower chamber at 37 °C and 5% CO 2 . After 6 h, cells that migrated to the bottom well of the transwell chamber were fixed in paraformaldehyde (Thermo Scientific) and stained with DAPI for quantitation. The chemotactic index is the ratio of migrated Mps to total Mps. Quantitative RT-PCR analysis RNA was isolated from tissues and cells using the Trizol reagent (Invitrogen, Carlsbad, CA), and cDNA was synthesized by reverse transcription kits (Takara, Dalian, China). All mRNA expression levels were normalized by comparing them to the housekeeping gene GAPDH. All RT-PCR primers are listed in Supplementary Table 6 . Prediction of transcription-factor binding sites The fragment between −2,000 and ±500 bp of the transcription start sites of the CX3CR1 and VEGF gene from the UCSC genome browser database was analysed for putative Smad binding element (SBE) motifs in TRANSFAC version 10.2 using PWMSCAN [54] . A match score with a P value <5 × 10 −6 was considered to indicate a high-confidence binding site prediction. Chromatin immunoprecipitation (Chip) assays Chip assays were conducted with a Magna ChIPTM A/G chromatin immunoprecipitation kit (Millipore) according to the manufacturer’s protocol. In brief, RAW264.7 and THP-1 cells were stimulated for 24 h by TGFβ1. Cells were then cross-linked with formaldehyde (1% final concentration), and the pellet was lysed and sonicated to shear the chromatin into 200–1,000-bp fragments. The lysates were diluted using a chromatin dilution buffer. The chromatin extract was incubated with 10 μg of rat anti-Smad2/3 antibody (Abcam) or rat IgG (negative control) at 4 °C with rotation overnight, and the antibody–antigen–DNA complex was collected by protein G-agarose. The immunocomplexes were washed and the protein–DNA complexes were eluted, and then proteinase K was used to reverse the cross-linking of protein–DNA complexes to free up DNA. DNA was purified with the DNA purification kit (Promega), dissolved in elution buffer, and used for quantitative PCR analysis. The primers used for amplification of SBE-containing fragmentsof CX3CR1 and VEGF genes are listed in Supplementary Table 7 . Luciferase reporter assay Mouse macrophage cell line RAW264.7(ATCC TIB-71) and Human monocyte cell line THP-1(ATCC TIB-202) were tested every 3 months for mycoplasma contamination by performing a PCR on the cell supernatant. They were seeded into 24-well plates and grown to 70% confluence. Luciferase reporter or control empty vector plasmids were co-transfected with RPL-TK (internal plasmid) (20:1) into cells by using a lipofectamine 2000 transfection reagent (Invitrogen). Cells were cultured in a medium containing 1% FBS and lysed 24 h after transfection. The Ep3 antagonist L798106 (Cayman, 0.1–10 μmol) or TGFβ1 (Selleck, 10 ng ml −1 ) was used to treat cells overnight 16 h after transfection. Luciferase activities were monitored with a dual luciferase reporter assay kit (Promega). Plasmid construction Mouse Cx3cr1 promoter DNA fragments (−453 to 124 bp) and Vegf promoter DNA fragments (–1,216 to 399 bp) were amplified from mouse macrophage genomic DNA by PCR. The two promoter fragments were subcloned into pGL3 (Promega). The reporter with the insert of a fragment of −453 to 124 of CX3CR1 gene was named S3+S4. Mutations were introduced into the third (mS3) and fourth (mS4) SBEs of the CX3CR1 promoter by QuikChange site-directed mutagenesis (Stratagene, La Jolla, CA). Human CX3CR1 promoter DNA fragments (−196 to 107 bp) and VEGF promoter DNA fragments (−1,278 to 134 bp) were amplified and subcloned into the PGL3 vector for the reporter assay. The PCR primers for promoter subcloningare listed in Supplementary Table 8 . In vitro HUVEC fibrin gel bead assay Human vascular endothelial cells (HUVECs), from PromoCell (C-12200) were mixed with dextran-coated Cytodex 3 microcarriers (GE) at a concentration of 400 HUVECs per bead in 1.5 ml of EGM-2 medium (Clonetics, Walkersville, MD). Beads with cells were shaken gently at 37 °C and 5% CO 2 every 20 min for 4 h. After incubating, beads with cells were transferred to a T2 tissue culture flask (Corning) and left overnight in 5 ml of EGM-2 at 37 °C and 5% CO 2 . After that, beads with cells were washed three times with 1 ml of EGM-2 and re-suspended at a concentration of 200 cell-coated beads per ml with 2.5 mg ml −1 of fibrinogen (Sigma) and 0.15 units ml −1 of aprotinin (Sigma). Five hundred microlitre of fibrinogen/bead solution was added to 0.625 units of thrombin (Sigma) in one well of a 24-well tissue culture plate. The fibrinogen/bead solution was allowed to clot for 5 min at room temperature and then at 37 °C and 5% CO 2 for 20 min. One millilitre of EGM-2 (which contains 2% FBS) with or without 0.15 units ml −1 aprotinin was added to each well and equilibrated with the fibrin clot for 30 min at 37 °C and 5% CO 2 ; 10 6 macrophage cells were plated on top of the clot. Assays were terminated at day 7 for immunostaining and imaging [55] . PG extraction and analysis Hearts collected from mice 14 days after MI were homogenized, and 500 μl supernatant were used for PG extraction. Heart prostanoid metabolites were extracted and quantitated using liquid chromatography/mass spectrometry/mass spectrometry (LC/MS/MS) analyses. In brief, following internal standards (2 μl), 40 μl citric (1M) and 5 μl BHT were added to the sample and then strenuously vibrated with 1 ml solvent (normal hexane: ethyl acetate, 1:1) for 1 min. After centrifugation (6,000 g min −1 ) for 10 min, the supernatant organic phase was collected and dried under a gentle stream of nitrogen, dissolved in 100 μl 10% acetonitrile in water. Production was normalized to total protein. Isolation of human blood Mos Human peripheral blood mononuclear cells (PBMCs) were purchased from Zenbio and resuspended (10 6 cells/10 μl) in sorting buffer (2 mM EDTA, 0.5% BSA in PBS) and stained with anti-human antibodies (Biolegend) specific for anti-CD14 and anti-CD16. Stained cells were filtered (70 μm) and sorted on a BD FACSAria II cell sorter using appropriate colour compensation for correcting spectral overlap and autofluorescence. Isolated CD14 dim CD16 + Mos were used for subsequent experiments. Mo adoptive transfer For zymosan-induced peritonitis mouse model, Mo subsets were sorted from spleens of EP3 F/F and EP3 F/F Lys Cre mice, then labelled with cell proliferation dye eFluor 670 (eBioscience) and injected into C57/BL6 mice 6 h after zymosan challenge by tail vain. For MI model, Mo subsets were collected from CD45.2 + mice as previously described [10] , and injected into CD45.1 + mice on day 3 post MI. Infarcted hearts at day 6 post MI were dissected for preparation of single-cell suspension and flow cytometric analysis. Histological analysis The infacted hearts were collected at indicated time points and embedded in the paraffin. The sections (6 μm) were stained with hematoxylin–eosin and Masson trichrome (Sigma). IPP software was used to analyse the necrotic area or collagen density as described [56] . Isolation of neutrophils and function assay APC-conjugated antibody to CD11b (M1/70),PE-conjugated antibody to CD45(30-F11) and APC-CY7-conjugated antibody to Ly6G (1A8)were purchased from Biolegend. Neutrophils were sorted from injured hearts by FACS and calculated by FlowJo software (Tree Star, Ashland, Ore). Ly6G (ab25377) were purchased for immunofluorescence in mice heart after MI. For reactive oxygen species (ROS) measurement, purified neutrophils were loaded for 20 min at 37 °C with dichloro-dihydro-fluorescein diacetate (DCFH-DA). Cells were washed and then production of ROS was quantified via flow cytometry by measurement of DCF. To detect intracellular myeloperoxidase, 5 × 10 4 neutrophils were lysed with TBS containing 0.2% Triton X-100 (50 ml) and the myeloperoxidase activity was measured as previously described [57] . Statistics Prism software (GraphPad Prism version 5.0) was used for statistical analysis. Results are shown as mean±s.e.m. Two-tailed student’s t -testing and one- or two-way ANOVA with Bonferroni post-hoc analyses were used for comparisons between different groups. A P value less than 0.05 was considered significant. Sample sizes were designed with adequate power according to the literature and our previous studies. Randomization and blinding strategy was used whenever possible. Data availability All the data supporting the findings of this study are either included in the manuscript and its Supplementary Information Files, or can be obtained from the corresponding author upon reasonable request. How to cite this article: Tang, J. et al . Activation of E-prostanoid 3 receptor in macrophages facilitates cardiac healing after myocardial infarction. Nat. Commun. 8, 14656 doi: 10.1038/ncomms14656 (2017). Publisher’s note : Springer Nature remains neutral with regard to jurisdictional claims in published maps and institutional affiliations.